Complete experimental toolbox for alignment-free quantum communication Quantum communication employs the counter-intuitive features of quantum physics for tasks that are impossible in the classical world. It is crucial for testing the foundations of quantum theory and promises to revolutionize information and communication technologies. However, to execute even the simplest quantum transmission, one must establish, and maintain, a shared reference frame. This introduces a considerable overhead in resources, particularly if the parties are in motion or rotating relative to each other. Here we experimentally show how to circumvent this problem with the transmission of quantum information encoded in rotationally invariant states of single photons. By developing a complete toolbox for the efficient encoding and decoding of quantum information in such photonic qubits, we demonstrate the feasibility of alignment-free quantum key-distribution, and perform proof-of-principle demonstrations of alignment-free entanglement distribution and Bell-inequality violation. The scheme should find applications in fundamental tests of quantum mechanics and satellite-based quantum communication. Current implementations of quantum communication (QC) use photons as the carriers of qubits (quantum bits), the basic units of quantum information. This is due to the fact that photons, known as so-called 'flying qubits', are easy to transport from one location to another [1] . Photonic free-space QC has been demonstrated for distances of hundreds of kilometers [2] , a progress that could soon lead to satellite-based long-distance QC [3] , [4] , [5] , [6] . However, standard approaches to QC, for example, the one based on encoding qubits into the polarization of photons, require that all users involved have knowledge of a shared reference frame. For instance, in the bipartite scenario, the emitter and receiver, conventionally called Alice and Bob, must initially align their local horizontal ( H ) and vertical ( V ) transverse axes, and then keep them aligned throughout the transmission ( Fig. 1a ). This, in turn, requires the exchange of a large (strictly speaking, infinite) amount of classical information. This represents, in general, an extra technical overhead, which can impose serious obstacles in the particular situations where the users are very far apart from each other, the misalignment between their frames varies in time, or the number of users is large, for example [7] , [8] . In general, the lack of a shared reference frame inhibits faithful QC, because it is equivalent to an unknown relative rotation, therefore introducing noise into the quantum channel [8] . 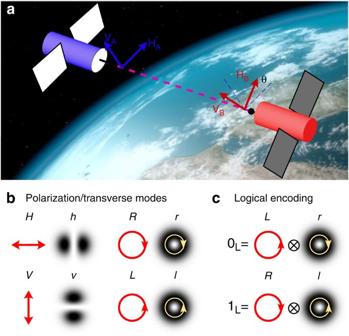Figure 1: Misalignment-immune single-photon qubits. (a) Alice and Bob, here depicted as satellites, need to carefully control the relative orientation between their horizontal (H) and vertical (V) axes to faithfully implement QC in free-space. Unknown misalignments around the propagation axis manifest as rotations of the transmitted qubits by unknown anglesθin theH−Vplane. (b) Qubits can be equivalently encoded in both polarization and transverse modes:H/Vdenote horizontal/vertical linear polarizations,L/Rleft/right circular polarizations,h/vhorizontal/vertical first-order Hermite-Gauss modes, andl/rleft- and right-handed first-order Laguerre-Gauss modes. TheL/Rpolarizations are eigenstates with eigenvalues ±ħ of the SAM, whereas thel/rmodes are the equivalent eigenstates of the OAM. (c) By combining SAM and OAM eigenstates of opposite handedness, two null-eigenvalue eigenstates of the total angular momentum arise. Both these hybrid states are invariant under rotations around the propagation axis, and can therefore encode misalignment-immune logical qubit states, called 0Land 1L. Figure 1: Misalignment-immune single-photon qubits. ( a ) Alice and Bob, here depicted as satellites, need to carefully control the relative orientation between their horizontal ( H ) and vertical ( V ) axes to faithfully implement QC in free-space. Unknown misalignments around the propagation axis manifest as rotations of the transmitted qubits by unknown angles θ in the H − V plane. ( b ) Qubits can be equivalently encoded in both polarization and transverse modes: H / V denote horizontal/vertical linear polarizations, L / R left/right circular polarizations, h / v horizontal/vertical first-order Hermite-Gauss modes, and l / r left- and right-handed first-order Laguerre-Gauss modes. The L / R polarizations are eigenstates with eigenvalues ±ħ of the SAM, whereas the l / r modes are the equivalent eigenstates of the OAM. ( c ) By combining SAM and OAM eigenstates of opposite handedness, two null-eigenvalue eigenstates of the total angular momentum arise. Both these hybrid states are invariant under rotations around the propagation axis, and can therefore encode misalignment-immune logical qubit states, called 0 L and 1 L . Full size image A possible solution to this problem is to exploit multi-qubit entangled states that are invariant under single-qubit rotations acting collectively on all the qubits (see refs 9 , 10 , 11 , 12 , 13 and references therein). These constitute particular instances of decoherence-free subspaces, originally introduced in the context of fault-tolerant quantum computing [14] , [15] , [16] , [17] . The idea is thus to encode logical qubits into rotationally invariant states of multiple physical qubits. These can, in principle, be realized with multiple photons [10] , [11] , [12] . However, the efficient production and detection of multi-photon states is a technological challenge, they are more susceptible to losses, and the requirement that multiple photons are subject to exactly the same rotation is very seldom perfectly satisfied. A more efficient way to circumvent misalignments is provided by exploiting multiple degrees of freedom of single photons [18] . In particular, the polarization and transverse spatial modes stand out for this purpose ( Fig. 1b ). Just as the circular polarization states are eigenstates of the spin angular momentum (SAM) of light, the helical-wavefront Laguerre-Gaussian modes are eigenmodes of its orbital angular momentum (OAM). The OAM degree of freedom is attracting a growing interest for applications in both classical and quantum photonics [19] , [20] , [21] , [22] . The peculiarity of the SAM and (first order) OAM eigenstates together is that, as they are defined with respect to the same reference frame, they suffer exactly the same transformation under coordinate rotation. Therefore, they satisfy the collective rotation requirement exactly, constituting an ideal pair to carry rotationally invariant hybrid qubits (see Fig. 1c ). Here we experimentally demonstrate a complete toolbox for the efficient encoding and decoding of quantum information in such photonic qubits, suitable for alignment-free QC. The core of our toolbox is a liquid crystal device, named ' q -plate' [22] , [23] , that maps polarization-encoded qubits into qubits encoded in hybrid polarization-OAM states of the same photon that are invariant under arbitrary rotations around the propagation direction, and vice versa . In other words, the q -plate acts as a universal encoder/decoder, where 'universal' refers to the fact that it works for any qubit state. The q -plate used in the present work is the result of a very recent technological advance allowing for the manufacture of electrically tunable devices with topological charge q =1/2 (ref. 24 ). This is the first time such devices are exploited in the quantum regime. In addition, the toolbox requires no interferometric stability as in previous proposals [18] , [25] , and can be set entirely in a robust and compact unit that could easily be mounted in a small satellite, for instance. Furthermore, our universal-decoder set-up features a built-in filtering mechanism that maps a wide class of physical errors into losses instead of logical errors. We show that, owing to this mechanism, the scheme is robust also against misalignments around axes other than the propagation direction, as well as against other spatial perturbations. We demonstrate the potential of our method by performing a proof-of-principle misalignment-immune implementation of the single-photon Bennett–Brassard (BB84) quantum key-distribution (QKD) protocol [26] , entanglement distribution, and the violation of the Clauser-Horne-Shimony-Holt (CHSH) Bell inequality [27] . Hybrid logical qubit encoding Our logical qubit basis is defined by the hybrid polarization-OAM single-photon states Subscript 'p' denotes the polarization Hilbert space, spanned by the left- and right-handed circular polarization states | L 〉 p and | R 〉 p , respectively, which are eigenstates of the SAM operator along the propagation direction ( z axis) of respective eigenvalues and . In turn, subscript 'o' stands for the OAM bidimensional subspace spanned by the left- and right-handed first-order Laguerre-Gauss modes | l 〉 o and | r 〉 o , eigenstates of the OAM operator of respective eigenvalues and . Finally, subscript L refers to the logical subspace of zero total angular momentum along z . The latter is spanned by the two hybrid states (1), null-eigenvalue eigenstates of the total SAM+OAM operator . Because the total angular momentum operator is the generator of state rotations, states (1) are both invariant under arbitrary rotations around the z axis (on this issue, see also ref. 28 ). More specifically, in a physical rotation about the z axis by any angle θ , the circular polarization states and OAM eigenmodes acquire equivalent phase factors on their own: . However, for tensor-product combinations with opposite handedness as (1), the individual phases cancel each other and the composite states remain intact. As a consequence, because of linearity, any coherent superposition (or incoherent mixture) of the two logical states, that is, the entire logical subspace, is also immune to all possible reference-frame misalignments during the entire QC session. Universal encoder/decoder The experimental set-up used to encode and decode arbitrary hybrid qubit states in the logical basis (1) is shown in Fig. 2 . The q -plates are liquid crystal devices that produce a spin-orbit coupling of the polarization and OAM contributions to the total angular momentum of photons [23] , [22] . The q -plate is a birefringent slab having a uniform optical retardation δ and a suitably patterned transverse optical axis, with a topological singularity of charge q at its centre. A 'tuned' q -plate with δ = π transfers quanta of angular momentum between the SAM and the OAM. Specifically, each photon suffers a variation in its OAM by an amount determined by the charge q and the SAM of the input polarization. q -plates with q =1 have been recently used to demonstrate interesting spin-OAM quantum information manipulations [29] , [30] , [31] , [32] , [33] . 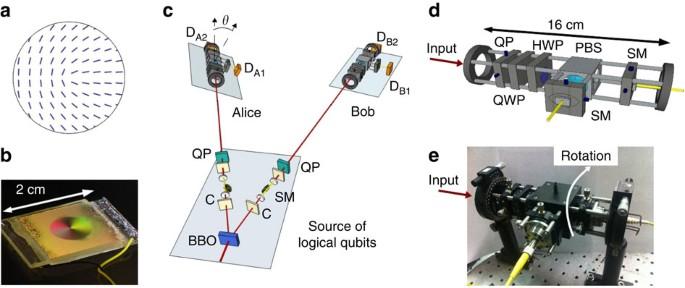Figure 2: Toolbox for experimental alignment-free quantum communication. (a, b) The liquid crystalq-plate with topological chargeq=1/2 works as a universal logical-qubit encoder/decoder. Panel (a) shows theq-plate optical axis pattern, whereas panel (b) is a photo of the device seen through crossed polarizers, under oblique illumination; different colours result from different optical axis orientations. Theq-plate birefringent retardation is electrically tuned. (c) Experimental set-up, in the configuration used to generate entangled rotationally invariant photon pairs and to perform a misalignment-immune demonstration of non-locality. Reference-frame misalignments are implemented by physically rotating Alice's entire measurement station around the optical axis by an angleθ. For the alignment-free BB84 QKD test, the entangled-photon source, together with Bob's measurement station, is taken as the transmitting party, and Bob's photon is used to herald the transmission of the other photon to Alice. The communication distance was 60 cm. (d) Schematics of the rotating device for measuring rotationally invariant qubits in arbitrary reference frames. (e) Photo of the actual measurement device. QP,q-plate; C, walk-off compensation crystals; SM, single-mode fibres; D, single photon detectors; HWP, half-wave plate; QWP, quarter-wave plate. Figure 2: Toolbox for experimental alignment-free quantum communication. ( a, b ) The liquid crystal q -plate with topological charge q =1/2 works as a universal logical-qubit encoder/decoder. Panel ( a ) shows the q -plate optical axis pattern, whereas panel ( b ) is a photo of the device seen through crossed polarizers, under oblique illumination; different colours result from different optical axis orientations. The q -plate birefringent retardation is electrically tuned. ( c ) Experimental set-up, in the configuration used to generate entangled rotationally invariant photon pairs and to perform a misalignment-immune demonstration of non-locality. Reference-frame misalignments are implemented by physically rotating Alice's entire measurement station around the optical axis by an angle θ . For the alignment-free BB84 QKD test, the entangled-photon source, together with Bob's measurement station, is taken as the transmitting party, and Bob's photon is used to herald the transmission of the other photon to Alice. The communication distance was 60 cm. ( d ) Schematics of the rotating device for measuring rotationally invariant qubits in arbitrary reference frames. ( e ) Photo of the actual measurement device. QP, q -plate; C, walk-off compensation crystals; SM, single-mode fibres; D, single photon detectors; HWP, half-wave plate; QWP, quarter-wave plate. Full size image A tuned q -plate with topological charge q =1/2 gives rise to the following transformations: where |0〉 o denotes a zero-OAM state, such as the fundamental Gaussian mode (TEM 00 ). We note that the radial profile of the | l 〉 o and | r 〉 o states generated by the q -plate is not exactly Laguerre-Gauss (see Methods for more details), but this does not affect their pure OAM-eigenstate rotational behaviour [22] . Indeed, the q -plate is ideally a unitary device (our q -plate was uncoated and had a transmission efficiency of about 85%), but the induced radial-mode effects (see Methods) may introduce about 40% of total additional losses in the final recoupling to the single-mode fibre before detection. Consider then a generic polarization-encoded qubit prepared in the TEM 00 spatial mode. From transformations (2), sending the qubit through the q -plate yields That is, the qubit is now encoded into the desired rotationally invariant space spanned by logical basis (1). Remarkably, the same q -plate device works also as a universal decoder, transferring generic rotationally invariant qubits to their polarization-encoded counterparts. Explicitly, by injecting |ψ〉 L into the q -plate, one obtains that can then be coupled into a single-mode fibre and analysed in polarization using standard methods. The measurement device is sketched in Fig. 2d . Again from the linearity of quantum mechanics, the encoding and decoding transformations (3) and (4) hold, even if the polarization state is part of some larger entangled state. In addition, an outstanding feature of the q -plate is that it realizes the polarization-transverse-mode coupling in a single compact device that requires no interferometric stability, therefore providing the scheme with a built-in robustness. Our first step was to experimentally verify that the encoding/decoding apparatus works properly in the case of stationary aligned reference frames. We prepared the input photon in one of the polarization states . The qubit was then mapped by a first q -plate into the rotationally invariant encoding, transmitted through free space to the measurement stage, then decoded back to polarization by a second q -plate, and finally analysed in polarization using a set of wave plates and a polarizing beam splitter (PBS). The full experimental apparatus is described in the Methods. The average measured fidelity with the input states was F =(98±1)%, indicating that the devices work nearly perfectly. Alignment-free quantum key distribution To experimentally demonstrate that the present QC set-up works well for arbitrary relative alignment of Alice and Bob's transverse reference frames, we mounted the q -plate, waveplates, PBS and optical fibre couplers in a compact and robust detection stage that can be freely rotated by any angle θ around the light propagation axis, as shown in Fig. 2d,e . Then, using heralded single photons, and for different angles θ , we encoded, transmitted and decoded, the four hybrid-qubit states required for the BB84 QKD protocol [26] : |0〉 L ,|1〉 L , and . We quantified the potential of our set-up for QKD by measuring the fidelities of the states prepared and measured with the ideal ones, as well as the qubit-error rates [34] and for the logical bases and , respectively. The experimental results are reported in Fig. 3a,b . 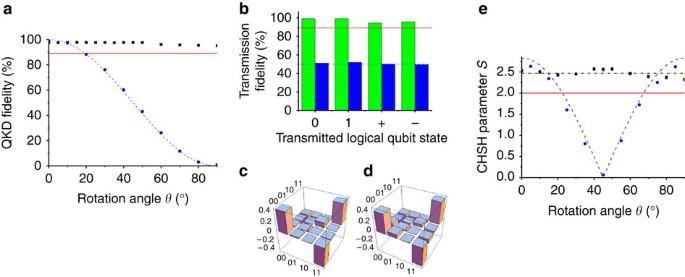Figure 3: Experimental results of alignment-free QC tests. (a,b) Measured fidelity of qubits encoded in the rotationally invariant polarization-OAM space, in a test of the BB84 quantum key distribution protocol, compared with that of standard polarization-encoded qubits. Panel (a) shows the fidelityFQKD(black square dots) averaged over the four hybrid qubit states used in the protocol, as a function of the misalignment angleθbetween the transmission and detection reference frames. Panel (b) shows the individual fidelity of each of the four states (green bars) observed over the whole QC session including all the different rotation angles probed. The latter accounts for the general situation where the misalignment could vary randomly between transmitted photons. In both panels, the blue dots/bars and dashed lines give, respectively, the measured and theoretically calculated fidelity for the standard case of polarization encoding. The red line delineates the QKD security threshold. (c,d) Quantum state tomography of the entangled state of hybrid qubits distributed between Alice and Bob, for the case of aligned reference frames (c) and for a misalignment ofθ=45° (d). In both cases, only the real part of the density matrices is shown, as the imaginary part is negligible. (e) CHSH parameterS(black squares) in experimental non-locality tests on photon pairs entangled in the rotationally invariant qubit space, as a function of the relative misalignmentθbetween Alice's and Bob's frames. The red line is the local-hidden-variable bound. The blue dots represent the measured values ofSfor the bare polarization-entangled states without the logical protection, whereas the blue dashed line is the theoretically calculated maximal CHSH parameter that would be obtained with pure maximally entangled polarization states. The black dot-dashed line, in turn, represents the overall CHSH valueSof the entire test, taking into account all the experimental runs with differentθ. Error bars result from Poissonian statistics. When not visible, the error bar is smaller than the symbol. Figure 3: Experimental results of alignment-free QC tests. ( a , b ) Measured fidelity of qubits encoded in the rotationally invariant polarization-OAM space, in a test of the BB84 quantum key distribution protocol, compared with that of standard polarization-encoded qubits. Panel ( a ) shows the fidelity F QKD (black square dots) averaged over the four hybrid qubit states used in the protocol, as a function of the misalignment angle θ between the transmission and detection reference frames. Panel ( b ) shows the individual fidelity of each of the four states (green bars) observed over the whole QC session including all the different rotation angles probed. The latter accounts for the general situation where the misalignment could vary randomly between transmitted photons. In both panels, the blue dots/bars and dashed lines give, respectively, the measured and theoretically calculated fidelity for the standard case of polarization encoding. The red line delineates the QKD security threshold. ( c , d ) Quantum state tomography of the entangled state of hybrid qubits distributed between Alice and Bob, for the case of aligned reference frames ( c ) and for a misalignment of θ =45° ( d ). In both cases, only the real part of the density matrices is shown, as the imaginary part is negligible. ( e ) CHSH parameter S (black squares) in experimental non-locality tests on photon pairs entangled in the rotationally invariant qubit space, as a function of the relative misalignment θ between Alice's and Bob's frames. The red line is the local-hidden-variable bound. The blue dots represent the measured values of S for the bare polarization-entangled states without the logical protection, whereas the blue dashed line is the theoretically calculated maximal CHSH parameter that would be obtained with pure maximally entangled polarization states. The black dot-dashed line, in turn, represents the overall CHSH value S of the entire test, taking into account all the experimental runs with different θ . Error bars result from Poissonian statistics. When not visible, the error bar is smaller than the symbol. Full size image Figure 3a shows the average fidelity F QKD over the four states, as a function of θ . F QKD is constantly above the value F T =89%, which corresponds to the well-known Shor-Preskill security proof threshold [35] . Above this, under the usual assumptions that Alice's source emits (logical) qubits, Bob's detectors perform (logical) qubit measurements, and there is no basis-dependent flaw in Alice's and Bob's systems [36] , unconditional security can be guaranteed. In contrast, the fidelity attained using polarization-encoded qubits falls below the security bound for angles θ >20°, even in the ideal noiseless case (blue dashed line). Figure 3b, in turn, shows the fidelity for each state, obtained by uniformly mixing the data over all measured angles θ . Again, all the individual-state fidelities are consistently larger than the security threshold. Indeed, the measured qubit-error rates, estimated as 1− F , were and , from which we expect a high secret-key fraction r =(70±1)% (ref. 34 ). Alignment-free entanglement distribution To test entanglement distribution, the photon pair is prepared in the polarization entangled state , where the superscripts A and B refer to Alice's and Bob's photons, respectively. The photons are coupled into single-mode fibres that select only states with zero OAM (TEM 00 mode). A q -plate at the output of each fibre transforms the polarization-entangled state to the rotationally invariant entangled state: To verify the generation of hybrid entanglement, we performed quantum state tomography of the experimental density matrix measured without misalignment ( θ =0). The tomographically reconstructed matrix, in the basis , is shown in Fig. 3c . The fidelity with the experimental polarization entangled state input to the encoder is , while the entanglement of , as given by the concurrence, is C =(0.85±0.03). As a first test on the rotational invariance of the state produced, we repeated the tomographic reconstruction with Alice's measurement stage rotated by θ =45°. The corresponding reconstruction is shown in Fig. 3d . The fidelity with is , and the concurrence is C =(0.84±0.03), consistent with the case θ =0. This indicates that our entanglement distribution scheme is immune to relative misalignments of Alice and Bob. Alignment-free quantum non-locality With the hybrid entangled state (5), we performed a violation of the CHSH inequality > in an alignment-free setting. In the inequality, a x and b y , with possible values 0 or 1, are the outcomes of Alice's and Bob's measurement settings x and y , respectively, with x and y equal to 0 or 1. Correlators , with 〈〉 the statistical average, quantify the fraction of events where Alice's and Bob's outcomes are observed to coincide. Any local-hidden-variable model satisfies the inequality [27] . For the rotationally invariant quantum violation of the inequality we chose the following hybrid measurement bases: {|0〉 L ,|1 L 〉} and {|+〉 L ,|−〉 L }, corresponding to Alice's settings x =0 and x =1, respectively, and and , corresponding to Bob's settings y =0 and y =1, respectively. Figure 3e reports the measured CHSH parameter S versus the rotation angle θ of Alice's measurement frame. The figure shows that the local-hidden-variable bound is violated for all angles, in striking contrast with the experimental polarization state (blue circles), or even with the ideal maximally entangled polarization state (blue dashed line). For the logically encoded states, we mixed the data of all different values of θ to test the violation's immunity to arbitrarily varying frame orientation, obtaining a value of S =(2.47±0.01)>2. This alignment-free extraction of non-local correlations reconfirms the rotational invariance of the quantum resources created here. Robustness of rotational-invariant hybrid qubits A remarkable feature of our polarization-OAM hybrid-encoding QC scheme is that it turns out to be robust against the spatial-mode perturbations arising in beam misalignments around axes other than the optical one and atmospheric turbulence effects. Such robustness appears at first glance counterintuitive, because the encoding involves the use of OAM, which is quite sensitive to all the above-mentioned spatial perturbations [37] , [38] (although significant progresses in pure OAM-based classical and quantum communication through the atmosphere have been recently reported [39] , [40] , [41] ). The main reason for such robustness is that the OAM spread induced by spatial-mode perturbations is neutralized by the polarization degree of freedom, which is in contrast very robust against those spatial-mode perturbations. This allows one to filter out, in the receiving unit, most components of the state that would otherwise decrease the fidelities. That is, the particular decoding set-up used intrinsically implements an effective quantum error-correction procedure that discards (but does not correct) all states outside the logical subspace. Indeed, spatial-mode perturbations will alter a generic hybrid qubit , transforming it into the following state: where | m 〉 o denotes a generic mode with OAM eigenvalue and C m,m ′ are the probability amplitudes for the photon OAM to be shifted from to , owing to the perturbation. However, in the decoding unit, the photon undergoes another q -plate transformation followed by a projection onto an m =0 Gaussian spatial mode (for example, by coupling it into a single-mode fibre), which leads to the following final state: Therefore, if the spatial-mode perturbation satisfies the condition the final polarization-encoded qubit will be identical to the initial one, except for a global phase and amplitude, and the communication fidelity will be preserved (in this simple analysis, we did not consider the radial modes; see Methods for a complete theory). In particular, every beam transformation that is mirror-symmetric with respect to a plane containing the initial beam axis will be symmetrical in the sign of OAM and hence will satisfy equation (9). For example, beam parallel displacements, tilts, elliptical deformations, or aperturings with a circular iris (even if off centre) or a half-plane mask (knife-edge), all have this symmetry. An axial misalignment, that is, a misalignment around an axis other than the optical one, between the transmitting and receiving communication units is equivalent to a beam translation and/or tilt, with both contained in the same plane, and can be treated analogously. Only symmetry-breaking combinations of two or more of the above effects may affect the fidelity. For example, a beam tilt combined with a beam displacement along a different plane will break the mirror symmetry and hence might introduce some degree of qubit alteration. (See Supplementary Methods for an explicit analysis of these beam-misalignment perturbations. [42] ) Also, the main optical effects arising from atmospheric turbulence, such as beam wandering and spreading are mirror-symmetric, so that the extent of qubit alteration is expected to be much less significant in our communication scheme than in the case of pure OAM communication. Another important class of transformations that satisfies equation (9) is that mathematically defined by pure multiplicative factors acting on the optical field, for example, the transformations arising from crossing any arbitrary inhomogeneous medium that is thin as compared with the Rayleigh length. It is easy to verify that these will be described by coefficients C m,m′ that depend on the difference m − m ′ and on the absolute values | m | and | m ′|, so that equation (9) is automatically satisfied. Weak turbulence, introducing only pure phase wavefront distortions, falls within this class of transformations and is therefore predicted to leave the qubit fidelity intact [37] . If we now consider the fact that light propagation in homogeneous media leaves the various OAM components constant, we conclude that equation (9) is satisfied even if the turbulent medium is followed and/or preceded by a long-distance free-space propagation, as in the case of earth to satellite (and vice versa ) communication through the atmosphere. Experimental tests of rotational-invariant qubit robustness As a first test, we considered transmission through two types of transverse apertures: a half-plane movable obstruction (knife) covering a variable fraction of the transverse mode, and an iris (or pinhole) with variable radius. We have measured the state transmission fidelity F for different input states, at both aligned and 45°-rotated measurement stages, with respect to the transmitting unit, and for an increasing disturbance due to the obstruction. The experimental set-up used for this test is illustrated in Fig. 4a . We encoded different polarization qubits using two wave plates and mapped them into the hybrid encoding using a q -plate. For the purpose of comparison, we also switched to a pure-OAM encoding by inserting a fixed linear polarizer after the q -plate, so as to erase the polarization content of the qubit. Then, the photon was sent through the obstruction and to the receiving unit, and the communication fidelity was measured as a function of the obstruction transmittance, by varying the aperture of the pinhole or the transverse position of the knife. Thus, the lowest transmittivity corresponds to a tiny aperture of the pinhole (0.2 times the beam size), or to the almost complete coverage of the beam. All reported experimental fidelities were obtained by averaging over the six eigenstates of three mutually unbiased bases, therefore providing a good representative of the average fidelity over any input qubit state. The experimental results are reported in Fig. 4b,c . It is seen that the average fidelity of hybrid qubits is independent both of the transmittivity of the aperture and of the rotation angle of the measurement kit, with a global average of F =(98±1)% for the case of iris and F =(96±1)% for the knife. Moreover, in the former case the fidelity is not affected by the displacement of the pinhole off the beam axis. For comparison, we tested the resistance of qubits encoded only in the two-dimensional OAM subspace o 1 ={|+1〉,|−1〉}, that is, the same subspace used for the hybrid encoding. In this case, the fidelity remains high ( F =(97±1)%) only when the cylindrical symmetry of the modes is not perturbed, as for the centred iris, although for all other cases (non-centred iris or knife), the fidelity drops rapidly with decreasing transmission. 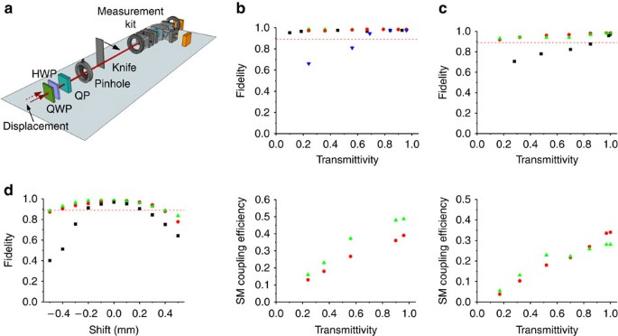Figure 4: Experimental results for rotational-invariant qubit robustness. (a) Experimental set-up adopted for the tests on the resistance of the rotational invariant hybrid photonic qubits to spatial-mode perturbations. In the schematics, we reported both the circular aperture (pinhole) and the half-plane obstruction (a movable knife-edge) that can alter the transmission of the qubits. Displaced beam is represented by a dashed red arrow. QP,q-plate; HWP, half-wave plate; QWP, quarter-wave plate. (b,c) Experimental resistance of rotational invariant hybrid qubits to beam perturbations, compared with the case of pure OAM qubits. Panel (b) refers to the case of circular aperture. Average fidelity of pure OAM qubits (black squares), hybrid qubits for a measurement stage rotated at an angleθ=0° (green triangles) and at an angleθ=45° (red circles) with respect to the transmitting unit. The blue triangles refer to the pure OAM qubits case, when the circular aperture is displaced off the beam axis by 5% of the beam waist (the hybrid qubit behaviour in the latter case was essentially indistinguishable from the centred aperture case). The transmission efficiency is determined by single-mode (SM) fibre-coupling efficiency after a circular aperture of varying radius, in the case of hybrid qubits only. Panel (c) refers to half-plane aperture. Average fidelities for hybrid qubits atθ=0° (green triangles) andθ=45° (red circles). Black squares are the corresponding results for pure OAM qubits. SM coupling efficiency after a movable half-plane aperture. (d) Experimental resistance of hybrid qubits (green triangles represent the caseθ=0° and red circlesθ=45°) to a beam displacement, compared with the case of pure OAM encoding (black squares). In all panels, the red dashed line delineates the QKD security treshold. The beam waist in our experiment isw0=(1.0±0.1)mm. Uncertainties are smaller than the symbols. Figure 4: Experimental results for rotational-invariant qubit robustness. ( a ) Experimental set-up adopted for the tests on the resistance of the rotational invariant hybrid photonic qubits to spatial-mode perturbations. In the schematics, we reported both the circular aperture (pinhole) and the half-plane obstruction (a movable knife-edge) that can alter the transmission of the qubits. Displaced beam is represented by a dashed red arrow. QP, q -plate; HWP, half-wave plate; QWP, quarter-wave plate. ( b , c ) Experimental resistance of rotational invariant hybrid qubits to beam perturbations, compared with the case of pure OAM qubits. Panel ( b ) refers to the case of circular aperture. Average fidelity of pure OAM qubits (black squares), hybrid qubits for a measurement stage rotated at an angle θ =0° (green triangles) and at an angle θ =45° (red circles) with respect to the transmitting unit. The blue triangles refer to the pure OAM qubits case, when the circular aperture is displaced off the beam axis by 5% of the beam waist (the hybrid qubit behaviour in the latter case was essentially indistinguishable from the centred aperture case). The transmission efficiency is determined by single-mode (SM) fibre-coupling efficiency after a circular aperture of varying radius, in the case of hybrid qubits only. Panel ( c ) refers to half-plane aperture. Average fidelities for hybrid qubits at θ =0° (green triangles) and θ =45° (red circles). Black squares are the corresponding results for pure OAM qubits. SM coupling efficiency after a movable half-plane aperture. ( d ) Experimental resistance of hybrid qubits (green triangles represent the case θ =0° and red circles θ =45°) to a beam displacement, compared with the case of pure OAM encoding (black squares). In all panels, the red dashed line delineates the QKD security treshold. The beam waist in our experiment is w 0 =(1.0±0.1)mm. Uncertainties are smaller than the symbols. Full size image As a second test, we performed a communication run while changing the angle of the measurement kit without reoptimizing the alignment of the single-mode fibre. This corresponds to introducing small uncontrolled tilt and displacements in the beam during the measurement. We found that the system preserves a good QC fidelity (that is, above the security threshold) for rotations up to 30°. Above this angle, it was necessary to slightly readjust the single-mode fibre alignment to restore a high fidelity. Finally, we tested the communication fidelity dependence on a controlled beam displacement, for two fixed angles of the measurement stage. Fig. 4d shows the behaviour of the average communication fidelity as a function of the beam displacement. The hybrid-qubit fidelity decreases with the displacement, but much slower than that of pure OAM encoding (see also the Supplementary Discussion ). QC has a fundamental role in the modern view of quantum physics and opens the possibility of a variety of technological applications. Uncontrolled reference-frame misalignments limit QC, as they turn the transmitted quantum messages into noisy, classical ones. Here we report the development of a robust and compact toolbox for the efficient encoding and decoding of quantum information into single-photon states that are invariant under arbitrary rotations around the optical axis. With this, all concerns on relative axis-orientation during quantum transmissions reduce simply to the basic requirement of establishing an optical link. Rotational invariance is achieved by exploiting decoherence-free subspaces spanned by hybrid polarization-OAM-entangled states. We experimentally showed the efficacy of these states through the feasibility demonstration of a cryptographic-key distribution protocol, distribution of entanglement, and violation of a Bell inequality, all in alignment-free settings. Importantly, as far as cryptographic security is concerned, our scheme does not introduce loopholes other than those already present in any photonic experiment with conventional encodings. We also emphasize that, even though the states used are themselves invariant only under rotations about the propagation axis, the scheme resists misalignments around other directions too. This is due to a filtering mechanism intrinsic to our universal-decoder set-up, which maps errors originating from beam rotations around axes other than the optical link, as well as other spatial perturbations, into signal losses instead of infidelity. Recently, interesting alignment-free approaches for QKD [43] and to extract non-local correlations [44] , [45] , [46] have been put forward. These, however, require that the relative axis orientations, though unknown, stay approximately static throughout the quantum data exchange session (see Supplementary Discussion for details). Remarkably, in contrast, our rotational-invariance protection works even if the relative orientations vary arbitrarily from measurement to measurement. Moreover, another important feature of the present scheme is that it does not restrict to non-locality and QKD but enables also fully general QC protocols, all misalignment-immune [18] . These include, for instance, quantum teleportation, dense coding, and entanglement swapping, the main ingredient of quantum repeaters. Finally, our scheme should find applications in the forthcoming experiments on long-distance satellite-based QC [3] , [4] , [5] , [6] . There, apart from misalignments, other issues may impose serious obstacles too, such as precise satellite laser-tracking, collection efficiencies, or finite-size effects (for QKD). However, immunity against arbitrarily varying transverse relative orientations not only solves for misalignments but also relaxes requirements on the repetition rates needed to overcome finite-size effects (see Supplementary Discussion ). Experimental apparatus The input photon pairs are generated via spontaneous parametric fluorescence in a β-barium borate (BBO) crystal cut for type-II phase matching, pumped by the second harmonic of a Ti:sapphire mode-locked laser beam with a 76-MHz repetition rate. The generated photons have wavelength λ =795 nm and spectral bandwidth Δ λ =3 nm, as determined by two interference filters. The spatial and temporal walk-off is compensated by inserting a λ / 2 wave plate and a 0.75-mm thick BBO crystal on each output mode [47] . The detected coincidence rate of the source is 8 kHz. The photons are delivered to the set-up via single-mode fibres, to define their transverse spatial mode to a pure TEM 00 , corresponding to OAM m =0. After the fibre output, two wave plates compensate the polarization rotation introduced by the fibre. The polarization-encoded photonic states are transformed into rotationally invariant hybrid states by q -plates with topological charge q =1/2. The average conversion efficiency of all the q -plates employed in the experiment has been optimized to (94±2)% by controlling the electric field applied to the device [48] , [49] . For the analysis of experimental data, we referred to the coincidence counts between detectors [ D A 1 , D B 1 ] and [ D A 2 , D B 2 ] shown in Fig. 2 , collected by a coincidence circuit with a gate of 3 ns. Typical coincidence rates were 30 Hz for the CHSH experiment and 300 Hz for the BB84 one. Theory of q -plate encoding/decoding with radial modes To fully describe the optical action of the q -plate, we need to consider both the azimuthal quantum number m , corresponding to the OAM eigenvalue in units of ħ, and a radial quantum number p . These two numbers can be defined, for example, as in the case of Laguerre-Gauss beams, although this is not the only possible choice and our treatment is general in this respect. We denote with | P , m , p 〉 the photon quantum state, including the spatial mode defined by m and p and the polarization state P (for example, L, R, H or V ). The q -plate transformation laws are as follows: where are coefficients that do not depend on the sign of m and m ′, owing to the mirror symmetry of the q -plate pattern. These coefficients can be also given explicit analytical expressions in a given radial basis (for example, the Laguerre-Gauss one), but these expressions are not needed for our purposes here. Let us now consider a generic input polarization-encoded qubit photon in a Gaussian mode TEM 00 ( m =0, p =0): After the q -plate, this photon is converted into the following rotation-invariant hybrid state (corresponding to the logical qubit): This generalizes the transformation (3), by including also the radial modes. In free-space propagation, the different spatial modes will acquire Gouy phase factors G | m|,p that depend only on the absolute value of m (see, for example, ref. 30 ). The final decoding procedure is based on a second q -plate followed by a spatial filtering into an output TEM 00 mode (that is, m =0, p =0; but the output radial basis need not be the same as the input one, as a different beam radius can be defined). This spatial filtering can, for example, be implemented by coupling into a single-mode fibre. This leads to the output polarization-encoded state , where Therefore | η | 2 gives the quantum efficiency of the encoding/decoding process. After decoding, this output state is ready for detection or for further quantum processing. Effect of spatial-mode perturbations during propagation Let us now consider the action of generic spatial-mode perturbation acting on the photons during propagation, as defined by the following transformation laws: where are suitable complex-valued coefficients (when ignoring the radial modes, they correspond to the C m , m ′ coefficients used in equation (6)). We assume here that the perturbation does not affect the polarization state. The Gouy phase factors describing free-space propagation can be included in (14) without loss of generality. Let us now consider the effect of the perturbation (14) on the encoded qubit (12), which is transformed into the following state: Next, we apply again to this perturbed state, the transformations used in the decoding unit ( q -plate and TEM 00 filtering), obtaining the following final state The latter equation shows that the qubit state will be unaffected, except for a global amplitude and phase factor, if and only if the following equality holds true: for all values of the radial indices p , p ′, thus generalizing equation (9). In other words, any spatial-mode perturbation that satisfies equation (17) will not alter the qubit transmission fidelity, although it may affect the transmission efficiency by increasing the photon losses. Explicit examples of spatial transformations arising in typical beam misalignment effects, such as beam translations and/or tilting, are considered in the Supplementary Methods . How to cite this article: D'Ambrosio, V. et al . Complete experimental toolbox for alignment-free quantum communication. Nat. Commun. 3:961 doi: 10.1038/ncomms1951 (2012).